Thermal transport in phononic crystals and the observation of coherent phonon scattering at room temperature Large reductions in the thermal conductivity of thin silicon membranes have been demonstrated in various porous structures. However, the role of coherent boundary scattering in such structures has become a matter of some debate. Here we report on the first experimental observation of coherent phonon boundary scattering at room temperature in 2D phononic crystals formed by the introduction of air holes in a silicon matrix with minimum feature sizes >100 nm. To delaminate incoherent from coherent boundary scattering, phononic crystals with a fixed minimum feature size, differing only in unit cell geometry, were fabricated. A suspended island technique was used to measure the thermal conductivity. We introduce a hybrid thermal conductivity model that accounts for partially coherent and partially incoherent phonon boundary scattering. We observe excellent agreement between this model and experimental data, and the results suggest that significant room temperature coherent phonon boundary scattering occurs. Almost all physical processes produce heat as a byproduct, making heat one of the most abundant forms of energy. Thermoelectric (TE) systems are among the few technologies that can convert heat directly into electricity, using the Peltier effect [1] . The performance of thermoelectric devices is gauged by the dimensionless thermoelectric figure of merit ZT =( S 2 σκ −1 ) T ; where S , σ , κ and T are the Seebeck coefficient, electrical conductivity, thermal conductivity and temperature, respectively. While Si-based semiconductors typically have very favourable power factors ( S 2 σ ) [2] , [3] , [4] , making them attractive for chip cooling and scavenging applications, their large phonon-dominated κ has prevented their use in TE systems. One approach is to use porosity to scatter phonons and hence reduce their contribution to κ [5] , [6] . However, there is a limit beyond which an increased porosity with corresponding small pore separation would lead to increased electron scattering and inadvertently reduce σ . Recently, it has been proposed that coherent boundary scattering in phononic crystals (PnCs) with relatively large feature sizes (≥100 nm) may hold the key to solving this problem by scattering phonons with minimal influence on electrons [7] , [8] , [9] . As phonons traverse such a lattice, they can undergo two types of scattering processes: simple particle-like incoherent scattering as a result of encountering a boundary, and wave-like coherent Bragg [10] scattering due to the periodic geometry of the artificial lattice of air holes. Here, coherence implies that the phonon phase is preserved and that scattering from material boundaries exhibits at least some measure of specularity. Practically, this can have profound implications because while incoherent boundary scattering depends only on the shape, size and separation of the holes, coherent boundary scattering additionally depends on the symmetry and geometry with which these holes are distributed. Thus, the existence of coherent scattering would enable further reduction of the thermal conductivity of the underlying material without the need for additional boundaries (for example, more air holes) by simply optimizing the PnC geometry. While coherent phonon boundary scattering has been observed at low temperatures (30–150 K) in 1D superlattices [11] , it has yet to be observed and verified in two-dimensional (2D) or three-dimensional (3D) PnCs, let alone at room temperature. Thus, the possibility of coherent phonon boundary scattering in Si-air PnCs at room temperature has generated widespread debate in the literature, given the relatively small wavelength of the phonon population dominating the thermal transport [6] , [8] , [12] , [13] , [14] , [15] . Experimentally, however, the thermal conductivity ( κ ) of PnC samples has consistently been measured to be significantly lower than that of an unpatterned film [6] , [7] , [9] , [14] , [15] , even after taking into account the combination of material removal and simple incoherent boundary scattering [7] , [9] , [14] . This suggests that another κ reduction mechanism, possibly coherent boundary scattering, must be taking place. The controversy was heightened by the discovery that ∼ 50% of the thermal phonons in Si have mean-free paths (MFPs) from 100 up to 1 μm [16] , which was recently verified experimentally [17] . Since it is logical to assume that a phonon remains coherent over its MFP, we suggest here that the MFP, rather than wavelength, should be used to determine whether or not a large enough fraction of the phonon population could travel sufficient distances while maintaining phase to experience the PnC lattice periodicity and thus undergo coherent boundary scattering. Several methods exist for calculating κ that assume partially coherent and partially incoherent phonon boundary scattering [6] , [8] , [12] , [14] , [15] . In particular, Hao et al. [12] , used Monte Carlo simulations combined with frequency-dependent phonon MFPs [16] to study phonon transport in a 2D square-lattice PnC, and concluded that phonon size effects caused by the periodic arrangement of the holes can be remarkable even when the hole size and spacing are much greater than the average phonon MFP. Tang et al. [6] suggested the possibility of a ‘necking effect’ for phonons with MFPs longer than the smallest dimension of the lattice. Dechaumphai et al. [18] used an approach where phonons with MFPs longer than the minimum feature size (distance between adjacent holes) were treated coherently as waves and were modelled using a finite-difference time-domain technique, while phonons with MFPs smaller than the minimum feature size were treated as particles and their transport modelled by the Boltzmann transport equation, taking into account only incoherent boundary scattering. Their study found some agreement with recent experimental work on nano-scale PnCs [9] , highlighting the importance of zone folding, however the model failed to reproduce the cross-plane data [7] possibly because of the lack of lattice periodicity in that direction. Conversely, Jain et al. [13] argued that a major deficiency in the previous models is their 2D nature, and proposed a full 3D model. Room temperature Monte Carlo simulations accounting for purely incoherent boundary scattering via the Boltzmann transport equation were used. The apparent agreement between theory and experiment [13] led the authors to conclude the absence of any coherent phonon boundary scattering. Although the incoherent nature of the model should have made it insensitive to propagation direction and scatterer geometry, the model was surprisingly deficient in reproducing the κ measured for unperforated slabs and the cross-plane PnC [7] direction, raising doubts that incoherent boundary scattering is solely responsible for the experimentally observed κ reduction in such PnCs. Thus, the matter of coherent versus incoherent phonon boundary scattering at room temperature remains an open question, and begs for a control experiment isolating the two scattering mechanisms to enables their independent quantification. In this communication, we focus on PnCs formed by the introduction of air holes in a Si matrix with minimum feature sizes >100 nm. To delaminate the incoherent and coherent phonon scattering mechanisms, we present an experiment that fixes the incoherent boundary scattering component and systematically varies the coherent component. We also introduce a hybrid thermal conductivity model that accounts for partially coherent and partially incoherent phonon boundary scattering, to enable the accurate prediction of thermal conductivity reduction in such structures. We observe excellent agreement between this model and the experimentally measured data, suggesting that significant room temperature coherent phonon boundary scattering does indeed occur. Theoretical framework Before describing the experiment presented in this work, we outline the theoretical framework for our approach. The phonon contribution to thermal conductivity in the structures of interest in this study can be modelled based on the Callaway–Holland formulation [19] , given by: where ℏ is the reduced Planck constant, f is a function accounting for the sample porosity ( φ ), q is the wavevector, ω ( q ) is the phonon dispersion, k B is the Boltzmann constant, T is the phonon temperature, v ( q )=∂ ω ( q )/∂ q is the phonon group velocity, τ ( q ) is the scattering lifetime of the phonons and the summation is over all phonon modes. In Si, the phonon scattering lifetime is dominated by umklapp, impurity and incoherent boundary scattering, which are given by [20] , and , respectively, where L is the effective sample length and is a measure of the average distance between boundaries [7] , [19] , [21] , [22] . The constants B , C , D and E measure the fractional influence of these different types of scattering mechanisms in a given sample, and are determined by fitting equation (1) to measured bulk Si data. Other thermal conductivity models highlighting different treatments of anharmonic umklapp phonon scattering were also considered ( Supplementary Note 1 and Supplementary Fig. 1 ). In highly porous samples, L can be replaced by the sample minimum feature size or critical dimension L c [5] , [6] ( Fig. 1 ), which corresponds to the maximum possible incoherent boundary scattering, or the incoherent scattering limit. 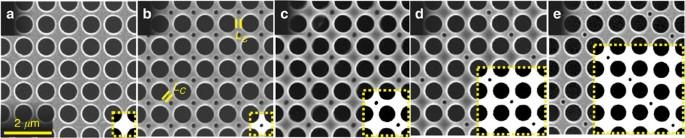Figure 1: SEM image of the fabricated PnC structures. All samples were fabricated to have a periodicitya=1,100 nm, thicknesst=366 nm and a chosen critical dimensionLc=250 nm. Highlighted in white is the unit cell of each supercell lattice: (a) SC, (b) 1 × 1, (c) 2 × 2, (d) 3 × 3 and (e) 4 × 4. The three scattering times are related to the total phonon scattering life time in equation (1) via Matthiessen’s rule: Figure 1: SEM image of the fabricated PnC structures. All samples were fabricated to have a periodicity a =1,100 nm, thickness t =366 nm and a chosen critical dimension L c =250 nm. Highlighted in white is the unit cell of each supercell lattice: ( a ) SC, ( b ) 1 × 1, ( c ) 2 × 2, ( d ) 3 × 3 and ( e ) 4 × 4. Full size image In this formulation, assuming a sufficiently large sample thickness [23] , [24] , [25] , [26] and feature sizes [13] , if coherent boundary scattering were absent, the Si phonon dispersion would remain basically unaltered before and after the PnC patterning and fixing L c would lead to a constant incoherent boundary scattering limit ( Supplementary Table 1 ). We thus set out to realize an experiment where the geometry of the PnC lattice is varied, while L c is kept constant. Previous electrical conductivity measurements on these and similar samples indicate that the impurity concentration remains practically unchanged before and after the PnC patterning [14] . The basis of our experiment is a PnC composed of a 2D simple cubic (SC) array of air holes in a Si slab with a designed periodicity a =1,100 nm, thickness t =366 nm and a chosen critical dimension L c =250 nm. Smaller interpenetrating holes, with dimensions chosen to keep L c constant, are then introduced at the center of the unit cell to create a series of lattices whose unit cell is now a composite supercell, as shown in Fig. 1 . These interpenetrating PnCs range from what is termed a 1 × 1 supercell, where the smaller hole is introduced at the center of every SC unit cell, to a 4 × 4 supercell that has four smaller holes added per every 16 SC unit cells. With this arrangement, the 1 × 1 supercell lattice has a unit cell size equal to that of the SC lattice but with the added smaller hole at the center, while the various n × n supercell lattices have unit cell sizes that are n 2 -times ( n =1, 2, 3, 4) that of the SC lattice. Thus, if phonon coherence persists through the scattering process, the Brillouin zone length of an n × n supercell is n -times smaller when compared with that of the original SC lattice, yielding n -times folded dispersion. This is real folding, brought about by the actual periodicity of the underlying lattice (see Fig. 2 ), as opposed to artificial folding created by choosing an arbitrarily large unit cell when calculating its dispersion. Fig. 2 shows the computed phonon dispersion normalized with the transverse wave speed ( c t ) using the plane wave expansion technique [8] . Implicit in this calculation is the assumption that phase information is retained throughout the entire spectrum. Examining Fig. 2 , it is clear that there is considerable deviation among the bands of the various supercell lattices, ranging from increased band curvature to band movement and even the introduction of new bands. To this extent, if these dispersions were to be theoretically unfolded, the various supercell bands would not overlay one another. This means that if coherent scattering is indeed taking place, there would be substantial deviation in group velocity and the density of phonon states across the various supercell lattices. This would manifest itself as a measurable systematic difference in κ as n increases that exceeded the combined influence of incoherent boundary scattering and the added porosity resulting from the introduction of the smaller holes. 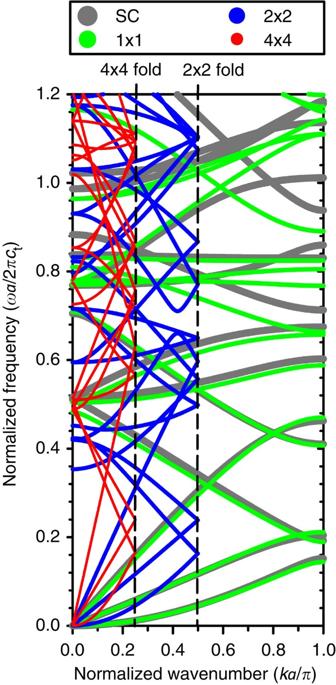Figure 2: Coherent zone folding due to PnC patterning inFig. 1. Plane wave expansion (PWE) calculated dispersions for the variousnxnsupercell lattices: SC (grey), 1 × 1 (green), 2 × 2 (blue) and 4 × 4 (red). The 3 × 3 supercell lattice was intentionally left out for clarity. The black dashed lines represent the respective Brillouin zone edges. Figure 2: Coherent zone folding due to PnC patterning in Fig. 1 . Plane wave expansion (PWE) calculated dispersions for the various n x n supercell lattices: SC (grey), 1 × 1 (green), 2 × 2 (blue) and 4 × 4 (red). The 3 × 3 supercell lattice was intentionally left out for clarity. The black dashed lines represent the respective Brillouin zone edges. Full size image Sample preparation and measurement Focused ion beam (FIB) milling with Ga ions ( Supplementary Methods ) was used to fabricate the PnC samples. Extreme caution was taken to avoid the contamination of the Si samples with any spurious Ga ions by using a sacrificial mask layer, which in addition to later etching of the samples resulted in the elimination of any added surface roughness due to the fabrication process (see the Methods section). The κ of various supercell samples was measured using a suspended island technique [27] ( Fig. 3 ), where a sample is mounted between two thermally isolated islands. By increasing the temperature of one island relative to the other and measuring the applied power and resulting temperature difference, the κ of the samples can be deduced [27] , [28] , [29] ( Supplementary Figs 2–4 ). Fabricated samples were attached to the suspended islands using a pick-and-place approach ( Supplementary Figs 5–6 ). Successive cuts using the FIB were employed to systematically calibrate out any unknown thermal resistances, and uniquely determine the thermal resistivity of the PnC supercell samples relative to that of an unpatterned Si slab of the same thickness. A detailed description of the process along with a quantification of the associated errors is given in the Supplementary Methods . 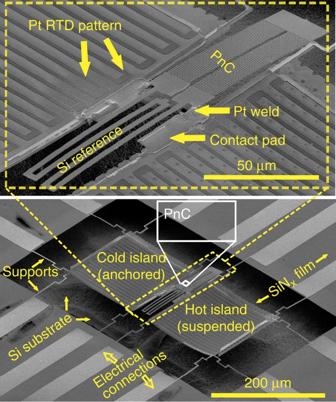Figure 3: SEM images of a measurement platform. This technique is used in this work for allκexperiments; RTD: resistive temperature detector. Figure 3: SEM images of a measurement platform. This technique is used in this work for all κ experiments; RTD: resistive temperature detector. 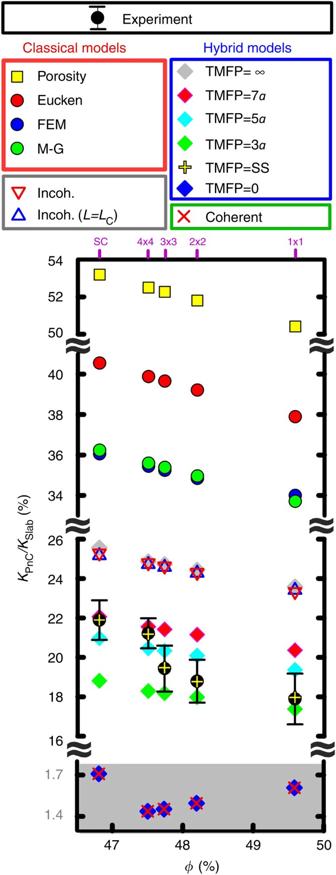Figure 4: Normalized thermal conductivities of PnC samples. The measuredκof the simple cubic (SC) and the 1 × 1, 2 × 2, 3 × 3 and 4 × 4 supercell PnC samples, along with the predicted values using various models described in detail in the text. Full size image Figure 4 shows a plot of the measured (black circles with error bars) κ of the various PnC lattices ( κ PnC ) of Fig. 1 normalized to that of an unpatterned Si slab ( κ Slab ) of the same thickness versus the sample porosity φ . A transition in the slope can be distinctively identified, suggesting a competition between two phenomena with opposing trends accompanied by a discrete transition. The results are compared with various theoretical model predictions ranging from simplistic porosity models to complex hybrid continuum-lattice dynamics models in order to explain the observed behaviour. Figure 4: Normalized thermal conductivities of PnC samples. The measured κ of the simple cubic (SC) and the 1 × 1, 2 × 2, 3 × 3 and 4 × 4 supercell PnC samples, along with the predicted values using various models described in detail in the text. Full size image Measurements versus traditional thermal conductivity models First, a series of classical mean-field models are evaluated. The yellow-squares represent the expected normalized κ due to simple material removal, obtained by using f ( φ )=1− φ . As expected, this severely underestimates the observed reduction in κ , as it neglects the pore (air hole) shape and surface area, accounting only for its volume. Analytical porosity models that take into account the added boundaries due to the pore shape and surface area are also evaluated. The red circles represent the results of the Eucken model [30] , while green circles represent those of the Maxwell–Garnett (M–G) model [31] f ( φ )=(1− φ )/(1+ φ ). Despite the complexity in the derivation of these models, they still largely underestimate the experimentally measured κ PnC reduction. This suggests that the reduction is not simply due to the porosity of the samples. Also shown on the plot are the results obtained from finite element method (FEM) simulations of the PnC samples using ANSYS [32] (blue circles). It is worth noting the excellent agreement between the M–G model and the FEM simulation results, lending more credibility to the M–G formulation over Eucken’s when accounting for porosity effects on the length scales considered here. Next, we include the effects of incoherent scattering by retaining the M-G factor in (1), using bulk Si dispersion, and accounting for the relative positions of the PnC boundaries (holes) through the choice of the value of L . One possibility is to simply use L c to ascertain the incoherent scattering limit (blue-triangles). Since this is the smallest physically-meaningful value of L , it corresponds to the maximum possible reduction from models assuming solely incoherent scattering and actually predicts a larger reduction in conductivity than that predicted by ref. 13 , which argues in favour of purely incoherent scattering. There, the effective sample characteristic length L eq is seen to be consistently larger than L c by more than 100 nm for each corresponding sample. However, the choice of L = L c treats all of the samples identically and is insensitive to the increase in the number of boundaries with the supercell order n . Thus, we also consider an alternate model for deducing an order-dependent sample size L . Noting that phonon scattering events by the in-plane air hole boundaries and the cross-plane sample surface boundaries are stochastic rather than mutually exclusive, a Matthiessen’s rule-type approach can be used to separate their influence as 1/ τ boundary, j =1/ τ cross-plane, j +1/ τ in-plane, j , with τ cross-plane, j = t / v j ( q ). The in-plane component can be evaluated using an order-dependent effective sample size L n , obtained by geometrically averaging over the relative in-plane boundary separations in a given sample [19] with τ in-plane, j = L n / v j ( q ) ( Supplementary Note 2 ). Alternately, each PnC sample can be viewed as a combination of n ( n-1 ) SC unit cells and n 1 × 1 unit cells. A boundary scattering lifetime associated with each type can then be calculated by averaging over the relative boundary separations in each unit cell and then combining using Matthiessen’s rule: 1/ τ in-plane, j =( n −1)/( nτ SC )+1/( nτ 1 × 1 ). The results of both approaches were found to be almost identical ( Supplementary Fig. 7 ) and are depicted by the red triangles in Fig. 4 . It is worth noting the agreement between the limiting case of L = L c and independently treating the in-plane and cross-plane incoherent scattering. Inspecting Fig. 4 , however, it is evident that even at maximum incoherent scattering the results still considerably underestimate the observed κ reduction in rate and magnitude and do not reproduce the slope transition, suggesting that an additional scattering mechanism with an opposing trend (increasing with n and decreasing with φ ) is possibly present. Consequently, the expected κ reduction was calculated assuming purely coherent (wave-like) phonon boundary scattering from the PnC holes, plotted as red-x’s in Fig. 4 . Here the PnC dispersion (a zoom-in of which is shown in Fig. 2 ) is used for ω ( q ), which implicitly accounts for the existence of the air holes; hence we set f ( φ )=1 in equation (1). Incoherent scattering from the surface boundaries of the sample was still accounted for by setting L = t . A total of over 46,000 modes were used in the calculation of the PnC dispersion [8] . It is worth noting here that this method is quite accurate for the acoustic phonon branches but to a lesser degree for the optical branches. However, the latter are estimated to contribute at most about 3.5% of the overall κ in bulk Si before any reduction [16] , [17] due to patterning. While our treatment clearly overestimates the reduction in κ due to the PnC patterning and exaggerates the dispersion effects of the PnCs on the acoustic branches, it is worth noting the reversal of the trend in κ PnC / κ Slab versus φ (and n ), consistent with our expectations based on Fig. 2 . Hybrid thermal conductivity model The results of these approaches indicate that a model that assumes partially coherent and partially incoherent boundary scattering is needed. The dilemma is in how to determine what portion of the phonon population undergoes coherent versus incoherent boundary scattering off of the PnC lattice holes. Since it is reasonable to expect a phonon to remain coherent over its MFP, one suggestion is to use the MFP to discern the scattering mechanism. We thus propose a model that incorporates frequency-dependent phonon MFPs in Si [16] , [17] and introduce the concept of a threshold-MFP (TMFP) that is essentially a measure of the phonon minimum coherence length. Phonons possessing a MFP above the designated TMFP value are able to sample the periodicity of the lattice and undergo coherent boundary scattering by the PnC, thus exhibiting a modified Si dispersion due to the PnC lattice, while phonons possessing a MFP below it do not ‘see’ the periodicity and thus undergo only incoherent boundary scattering and follow the unmodified Si dispersion. Therefore, the incoherent and coherent boundary scattering contributions to κ PnC are individually weighed by the fractional portion of the phonon population based on their MFPs with respect to the TMFP (See Supplementary Note 3 ). Given the absence of a direct way to experimentally measure the coherence length of phonons, we use the thermal conductivity measurement itself as a gauge for this determination. The TMFP is thus incorporated as a free parameter used to tune the model against the experimental measurements. While we acknowledge that a transition between coherent and incoherent boundary scattering should be gradual, there exists no practical theoretical foundation that allows us to gradually relax the preservation of the phonon phase as the mean-free path decreases (frequency increases) when we calculate the plane wave expansion-based PnC dispersion. The diamonds in Fig. 4 represent the results of five choices of the TMFP value. Note that our hybrid model correctly reproduces the limiting cases matching the purely coherent scattering calculation at TMFP=0 (blue-diamonds) and the incoherent scattering case at TMFP=∞ (grey-diamonds), including the reversal of the trends between both cases, thus lending credence to the model ( Supplementary Note 4 and Supplementary Fig. 8 ). It is particularly interesting that the hybrid model agrees well with the experimental data when the TMFP is large enough to cover 3–5 lattice periods, as this is similar to the literature-accepted bounds [10] , [33] , [34] , [35] , [36] , [37] , [38] , [39] for the fewest and largest number of periods needed to observe PnC behaviour. It is instructive to point out that the bounding TMFP values listed in Fig. 4 represent a population average over all supercell samples, which is a gross approximation as the TMFP is likely to be geometry (supercell) dependent. To this end, the yellow pluses in Fig. 4 represent the sample-specific TMFPs, designated TMFP-SS. Inspection of the TMFP-SS values ( Supplementary Note 4 and Supplementary Fig. 9 ) shows that the 1 × 1 supercell and the SC lattices are characterized by the smallest and largest TMFP-SS values respectively, and hence the largest and smallest respective fractions of coherently boundary scattered phonons. This is to be expected, since the 1 × 1 supercell lattice has the largest areal density of scatterers, and hence on average requires that phonons traverse much shorter distances before encountering a boundary scattering event as compared to the SC case. Thus on average, for coherent boundary scattering to occur, it would be necessary to conserve phase information over much shorter distances (shorter times) in the 1 × 1 case as compared with the SC case. Thus this condition is likely to be met by a larger fraction of phonons in the 1 × 1, and a comparatively much smaller portion of the phonon population in the SC case. Indeed, one can easily show that the number of equidistant scatters per unit cell is 4( n +1)/ n , in which case SC represents the limit as n →∞ and is consistent with Supplementary Fig. 7 . Furthermore, the location of the slope transition between the 4 × 4 and 3 × 3 experimental points can also be explained based on the calculated TMFP-SS values ( Supplementary Note 5 ). According to ref. 16 , which uses a density functional theory approach to study heat transport in Si, it is clear that there exist certain heavily-populated phonon modes that dominate over other less-populated ones [16] . More specifically, ref. 16 identifies several distinct MFP bands that result collectively in a nonlinear increase in the accumulation function; a range beyond 10 μm, and two bands starting around 7.9 and 4.3 μm that are of particular interest. Examining our reported TMFP-SS values, it is seen that the TMFP-SS for the 1 × 1, 2 × 2 and 3 × 3 supercells are about or <4.3 μm, while both the SC and 4 × 4 supercells are found to be much larger than that value (approaching 7 μm). Since by definition the TMFP-SS is the cutoff value per sample for the MFP beyond which a significant portion of the population undergoes coherent scattering, its value can be used to mark (on average) which of the dominant states the supercell phonon population predominantly belongs to or is influenced by. Striking correlation is observed in Supplementary Fig. 10 , suggesting that the 1 × 1, 2 × 2 and 3 × 3 supercells can be associated with the 4.3-μm band, while the 4 × 4 and SC supercells can be associated with the 7.9-μm band; thus proffering an explanation for the location of the experimentally observed slope transition. Finally, we wish to point out that while it is tempting to try to attribute the decrease in thermal conductivity of the supercell samples to the added surface boundaries of the interpenetrating holes, the added surface area is actually a false indicator of the effect of the added boundaries and would yield contradictory conclusions. This is explained in detail in Supplementary Note 6 . In this article, we present evidence that coherent scattering of phonons can indeed take place in 2D PnCs with submicron features including the first, to our knowledge, room temperature experimental observation of this phenomenon in such lattices. We also introduced the concept of a threshold mean-free path in conjunction with a hybrid theoretical model, where the incoherent and coherent contributions to thermal conductivity are weighted according to the fractional portion of the phonon population mean-free paths relative to that threshold. Although the periodicity of the PnC samples is large compared to the average phonon wavelength, our results indicate that a significant portion of the phonon population remains coherent even after undergoing several scattering events. From a different perspective, since there is no direct way to measure the coherence length, our approach has enabled us to use the thermal conductivity as a macroscopic metric for inferring the average phonon coherence length in our PnC samples. It is imperative to realize that the coherence length deduced here is an average over the total population, whereas the actual coherence length of individual phonons is likely both frequency and geometry dependent. Our results reinforce the suggestions of coherent phenomena indeed taking place in PnC samples, as postulated by Yu, et al. [9] and Dechaumphai, et al. [18] It also highlights the importance of accurately calculating the frequency-dependent phonon mean-free path, as presented in refs 12 , 13 . This work may hold the key to unprecedented TE performance through further suppression of phonon transport in porous samples with no added influence on electron propagation, by simply arranging the pores in an optimal PnC geometry. While the coherent PnC effects seen here represent a small yet significant fraction of the overall thermal conductivity reduction, their presence at room temperature is extremely encouraging. Given that a more pronounced effect is expected at lower temperatures, the impact on TE cooling could be profound. We point out that this PnC technology is applicable to all semiconductor materials, and could result in a net gain in ZT for any material that is limited by a large κ and that has a thermal conductivity that is dominated by phonon, rather than electron, transport. The realization of the aforementioned control experiment requires the ability to accurately control the fabricated PnC dimensions. To accomplish this, we used FIB milling with Ga ions ( Supplementary Fig. 11 ) to fabricate the supercells proposed in Fig. 1 . FIB milling of the phononic crystal samples To avoid obtaining erroneous results, three risks had to be addressed and mitigated, namely: (1) varying cross-sectional dimensions due to using a Gaussian beam of ions leading to uncontrolled variation of the porosity; (2) the uncontrolled implantation of Ga ions in and around the PnC holes and in turn an unquantifiable random impurity scattering; and (3) the added surface roughness and the thin damage ring of amorphous Si that is associated with milling of the air holes due to the sputtering and re-deposition of Si atoms. The first and second issues were completely eliminated by the use of a sacrificial mask layer of a material that has a lower sputtering yield than Si ( Supplementary Methods , and Supplementary Fig. 12 ). The fabrication process of the structures shown in Fig. 1 yielded near-vertical sidewalls with less than a 3° measured slant angle ( Supplementary Fig. 13 ). The average dimensional variation in L c was found to be about 5 nm. Furthermore, the use of a sacrificial layer coupled with sample postprocessing and etching removed almost all of the contaminating Ga ions. Supplementary Fig. 14 shows energy dispersive X-ray spectroscopy data at different acceleration potentials, revealing that the concentration of the remaining Ga ions is negligible and is on the order of the O-atoms present in the native surface oxide. Roughness considerations After sample post-processing, etching, and removal of the protective mask layer, a change in the surface roughness of the samples is not observed. Fig. 5 shows an atomic force microscope image of the sample’s top surface at various locations before and after the PnC patterning. Examining the figure, it is evident that r.m.s. (root mean square) roughness is not only comparable between pre- and post-fabrication unpatterned Si areas, but appears to decrease in the PnC and the post-fab Si regions. The other source of roughness is the PnC hole’s sidewalls. We inspected the PnC hole-sidewalls ( Supplementary Fig. 15 ) using high-resolution transmission electron microscopy (TEM) ( Supplementary Fig. 16 ). The measured r.m.s. roughness value at the boundary of the PnC holes was found to be ∼ 1 nm ( Supplementary Fig. 17 ). Details of this study ( Supplementary Note 7 ) and the effects of roughness ( Supplementary Note 8 , and Supplementary Fig. 18 ) are presented. 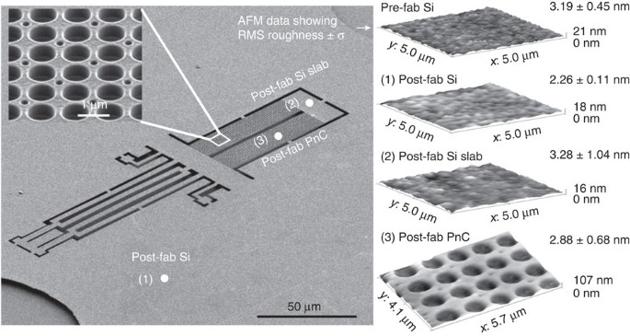Figure 5: PnC sample roughness characterization. SEM image (left) of a PnC—matrix sample and atomic force microscope (AFM) scans (right) of the Si surface pre-fabrication and post-fabrication demonstrating that the roughness of the Si surface did not statistically change during processing. All roughness measurements are RMS values. Figure 5: PnC sample roughness characterization. SEM image (left) of a PnC—matrix sample and atomic force microscope (AFM) scans (right) of the Si surface pre-fabrication and post-fabrication demonstrating that the roughness of the Si surface did not statistically change during processing. All roughness measurements are RMS values. Full size image Finally, the damage ring along the perimeter of the PnC hole due to FIB milling is removed during the final step of processing when HF acid is used to release the device [40] . In addition, it should be noted that the damage ring thickness is on the order of 10 nm [41] and is independent of the sizes of the holes or the beam dwell time. Measurements of the diameters of the holes were made after the removal of this damage ring. To verify the dimensions of the fabricated PnC samples, SEM images covering the entire area of each sample were taken. Image recognition software was then used to determine the average dimensions reported above. The result is in excellent agreement with the target dimensions, with a large hole diameters of 845 nm±6 nm, a smaller hole diameter of 211 nm±6 nm, and a critical length of 250 nm±5 nm. How to cite this article: Alaie, S. et al. Thermal transport in phononic crystals and the observation of coherent phonon scattering at room temperature. Nat. Commun. 6:7228 doi: 10.1038/ncomms8228 (2015).